Determination of nanoparticle size distribution together with density or molecular weight by 2D analytical ultracentrifugation Nanoparticles are finding many research and industrial applications, yet their characterization remains a challenge. Their cores are often polydisperse and coated by a stabilizing shell that varies in size and composition. No single technique can characterize both the size distribution and the nature of the shell. Advances in analytical ultracentrifugation allow for the extraction of the sedimentation ( s ) and diffusion coefficients ( D ). Here we report an approach to transform the s and D distributions of nanoparticles in solution into precise molecular weight ( M ), density ( ρ P ) and particle diameter ( d p ) distributions. M for mixtures of discrete nanocrystals is found within 4% of the known quantities. The accuracy and the density information we achieve on nanoparticles are unparalleled. A single experimental run is sufficient for full nanoparticle characterization, without the need for standards or other auxiliary measurements. We believe that our method is of general applicability and we discuss its limitations. Hybrid inorganic–organic core–shell nanoparticles (NPs) are finding a wide range of applications in solar cells [1] , optoelectronics [2] , [3] , nanophotonics/plasmonics [4] , catalysis [5] , [6] , [7] , drug delivery [8] , [9] and biomedical imaging agents [10] , [11] . Their chemical [12] , electronic [13] , optical [2] , [12] , [14] , magnetic [15] and catalytic [13] , [16] properties, and self-assembly [17] , [18] inherently depend on their size and composition. Hence, as industrial and research needs grow more complex, it becomes imperative to find a versatile, reliable and scalable method for the full characterization of these particles. The total evaluation of a NP entails a global analysis that pieces together measurements taken from multiple techniques ( Fig. 1 ). However, such an approach usually presents an incomplete picture of the sample in question since NPs are rarely perfectly monodisperse. Methods that characterize the organic shell give only macroscopic averages of the whole sample distribution, and size analysis techniques provide distribution data only of the total NP (see Fig. 1 ). Combined analyses are possible, but become challenging as the complexity (for example, polydispersity) of the sample increases. For example, the recent advances, where fractionation and size analysis are used in series, provide a wealth of information, but at the expense of numerous assumptions and laborious approaches [19] . Arguably, NP characterization has become a rate-limiting step, hindering the development and prospective uses of these promising materials. 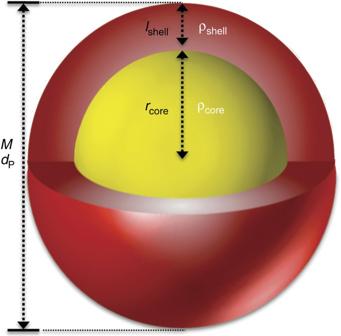Figure 1: Typical characterization schemes for core–shell nanoparticles. The core density (ρc) is normally taken as the bulk density47or quantified by x-ray diffraction assuming a conformation to a particular model. TEM, scanning transmission electron microscopy, and x-ray diffraction are the most commonly used methods to investigate core radius (rc) and composition; yet, these techniques provide little information on the organic ligand shell (due to the low contrast of organic material). Furthermore, core size distributions extracted from TEM images are generally skewed by the choice of the selected area of the sample, small sampling size (a few thousand particles at most) and the undercounting of the smallest particles (due to their low TEM contrast). To measure total particle diameter (dP), dynamic light scattering (DLS) is not particularly sensitive for small particles and atomic force microscopy (AFM) or scanning tunnelling microscopy (STM) are slow and share the same sampling selection limitations of TEM. Both size exclusion chromatography and gel electrophoresis require a standard. For small particles (<40 kDa), mass spectroscopy (MS), in particular electrospray ionization MS (ESI-MS), is the preferred method to measure particle molecular weight (M); but, problems in stability and complexity limit this technique33. To characterize the organic ligand shell density (ρL), thermogravimetric analysis can be utilized, but it is accurate only for a monodisperse species48. Nuclear magnetic resonance (NMR) can also provide information on the composition and density of the ligand shell, but counterions present a major problem, and again, the technique is limited only to large sizes49. No single technique can simultaneously measure all six parameters with a single experiment. Figure 1: Typical characterization schemes for core–shell nanoparticles. The core density ( ρ c ) is normally taken as the bulk density [47] or quantified by x-ray diffraction assuming a conformation to a particular model. TEM, scanning transmission electron microscopy, and x-ray diffraction are the most commonly used methods to investigate core radius ( r c ) and composition; yet, these techniques provide little information on the organic ligand shell (due to the low contrast of organic material). Furthermore, core size distributions extracted from TEM images are generally skewed by the choice of the selected area of the sample, small sampling size (a few thousand particles at most) and the undercounting of the smallest particles (due to their low TEM contrast). To measure total particle diameter ( d P ), dynamic light scattering (DLS) is not particularly sensitive for small particles and atomic force microscopy (AFM) or scanning tunnelling microscopy (STM) are slow and share the same sampling selection limitations of TEM. Both size exclusion chromatography and gel electrophoresis require a standard. For small particles (<40 kDa), mass spectroscopy (MS), in particular electrospray ionization MS (ESI-MS), is the preferred method to measure particle molecular weight ( M ); but, problems in stability and complexity limit this technique [33] . To characterize the organic ligand shell density ( ρ L ), thermogravimetric analysis can be utilized, but it is accurate only for a monodisperse species [48] . Nuclear magnetic resonance (NMR) can also provide information on the composition and density of the ligand shell, but counterions present a major problem, and again, the technique is limited only to large sizes [49] . No single technique can simultaneously measure all six parameters with a single experiment. Full size image NP research lacks a single platform that quickly, easily and completely characterizes the size, density (an indicator of composition) and molecular weight of each unique particle species among a heterogeneous mixture, with a single experimental measurement. However, recent 2D mathematical and computational modelling advancements in sedimentation-velocity analytical ultracentrifugation (SV-AUC) [20] allow for the mapping of sedimentation coefficient and diffusion coefficient distributions of species present in solution [21] , [22] . AUC is performed using an ultracentrifuge fitted with one or more optical detection systems, allowing the observation of the fractionation process of a species dissolved in solution. The sedimentation process is monitored by a scanning UV/VIS optical detection system that records the concentration profile, c ( r , t ), with respect to radial distance from the rotor ( r ) and time ( t ). The c ( r , t ) is subsequently numerically modelled and transformed into a sedimentation coefficient ( s ) and diffusion coefficient ( D ) distribution, c ( s , D ) [21] . SV-AUC is a tool particularly suited for the study of NPs [23] , [24] , [25] , [26] . First, the technique characterizes the sample in solution; hence it provides an opportunity to observe the properties in conditions similar to conditions present in most applications (for example, self-assembly, solution casting, physiological ... etc.). Second, because the data of an AUC experiment is analysed in the framework of fundamental thermodynamic principles [23] , it does not require any standard or calibration. Finally, AUC requires little sample (<1 mg) and minimal preparation and it encompasses virtually any particles soluble in a liquid phase. The presumed requirement for a priori knowledge of the density for the target species has always prevented wider implementation of AUC. This becomes an even greater hurdle in core–shell NPs, because their density depends on the ratio between the size of the core and that of the shell. Despite numerous attempts to circumvent the issue of direct NP density measurement to obtain quantitative AUC characterization [27] , [28] , the problem still exists, particularly for samples for which density depends on size (for example, particles with a fixed length shell but variable sized cores). Here we demonstrate a simple scheme to fully characterize NPs with 2D SV-AUC that not only overcomes the limitation of a priori density measurement, but also allows us to obtain the density distribution of a species, in addition to its size and molecular weight distributions. Our method is enabled by the simultaneous extraction of both the sedimentation and diffusion coefficient distributions from the sedimentation process of the NP species present in the sample. Our approach differs from other SV-AUC studies on NPs—including Svedberg's original experiments [25] , [26] —in that we require no prior measurement nor make any assumptions regarding the density of the NPs and that we utilize both the diffusion data (ignored or unavailable in most studies) and the sedimentation data obtained from 2D SV-AUC to determine NP density. It should be further noted that we assume a 1:1 correspondence between the hydrodynamic Stokes' diameter and the actual diameter of the particle, which we prove to be an accurate description for a wide range of NPs. As our methodology is simple, rapid, accurate and scalable, we expect the findings in this research article to be useful to anyone interested in the properties and applications of NPs. This method could become useful for those applications that are especially sensitive to NP size and overall variability. Theory The Lamm equation describes the evolution of a solute concentration distribution under centrifugation [23] , [29] : A solution to the Lamm equation is a spatially and temporally resolved concentration function, c ( r , t ), sigmoidal in shape, real-valued and differentiable. The analytical ultracentrifuge records experimental concentration profiles that satisfy the Lamm equation. Although the general Lamm equation is impossible to solve with a closed analytical solution [30] , modern computational software (such as SEDFIT [31] or Ultrascan [22] ) can directly fit approximate solutions of the Lamm equation to a set of experimental data points for an entire sedimentation process (for example, Supplementary Fig. S1 ). SEDFIT, used for this work, employs a numerical finite element method with an adaptive grid-size algorithm and moving frame of reference, which drastically improves diffusion modelling compared with other computational models and numerical solutions [20] . The numerical method analysis results in a high-resolution differential distribution of sedimentation coefficients c ( s ), a model that deconvolutes diffusion from sedimentation and reduces peak broadening. The c ( s ) model can be easily extended to include two-dimensional size-and-shape information, c ( s , D ) [21] . Finally, all peaks can be tested to ensure authenticity by Monte-Carlo analysis and F-statistics [32] . The basis for AUC's theoretical treatment is in thermodynamic and hydrodynamic principles [23] . During sedimentation velocity experiments, three forces act on a sedimenting solute. A centrifugal force induced by the acceleration of the rotor, ω 2 r , is proportional to particle mass, so that larger particles sediment faster than smaller ones (provided the mass of the particle is greater than the displaced mass of the solvent). The buoyant force (governed by the Archimedes' principle) and frictional force act in opposite direction to the centrifugal force, impeding sedimentation. The frictional force is generated by movement of the solute through the solvent according to the hydrodynamic treatment of viscous drag and is proportional to a frictional coefficient and the solute terminal velocity ( u ). The three forces come into balance very quickly (within ~10 −6 s [23] ) and the particle achieves terminal velocity. Rearrangement of the force balance yields the well-known Svedberg equation [23] : where the sedimentation coefficient, s , is defined as the solute terminal velocity per unit centrifugal field. Here ρ s is solvent density and is the partial specific volume, which can generally be equated with the inverse density of the particle (that is, ). For a smooth, compact sphere under the limit of low Reynolds number (that is, small size), Stokes' law and the Stokes-Einstein [23] relation combine to give D in terms of the hydrodynamic Stokes' diameter d H : where η s is the viscosity of the liquid and k b is Boltzmann's constant ( k b = R / N A =1.38065×10 −23 JK −1 ). Equations 2 and 3 are merged and rearranged to form the well-known expression providing the basis for measuring Stokes-equivalent spherical diameters with AUC [23] , [25] , [26] : In our treatment, we assume that the Stokes' diameter and the particle diameter are approximately equal (that is, d H = d P ), and combine Equations 3 and 4—and re-express Equation 2 in terms ρ P —to obtain formulas that allow us to determine the particle parameters ρ P , M , and d P in terms of the experimentally measured s and D value distributions: Equations 5a, 5b and 5c represent the theoretical basis underlying our 2D SV-AUC measurements. In contrast to most SV-AUC approaches where only Equation 5c is used by assuming a particle density ( ρ P ), we find that the ρ P can instead be calculated from s and D through Equation 5a. Our approach's accuracy at predicting the density ( ρ P ), molecular weight ( M ) and diameter of NPs ( d P ) is demonstrated experimentally in the next section. 2D AUC of single monodisperse standard nanoclusters As an illustrative test case, we first measured the 'magic-sized' NP Au 144 (SR) 60 ( R =−CH 2 CH 2 Ph) (synthesis [33] and ESI-MS characterization detailed in Methods). 2D SV-AUC was performed on a sample of Au 144 (SR) 60 nanoparticles (Experimental details provided in Methods). 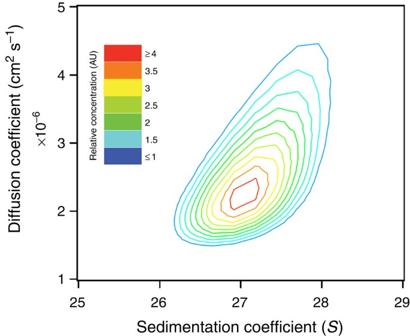Figure 2: 2D AUC distribution for Au144(SR)60nanoclusters. The sedimentation and diffusion coefficient distributions for the Au144(SR)60magic-sized nanocluster in toluene (T=20 °C). Figure 2 plots the analysis obtained from the data collected for the Au 144 (SR) 60 cluster. Figure 2: 2D AUC distribution for Au 144 (SR) 60 nanoclusters. The sedimentation and diffusion coefficient distributions for the Au 144 (SR) 60 magic-sized nanocluster in toluene (T=20 °C). Full size image The particle density was first calculated by Equation 5a using the integrated, weight-averaged diffusion and sedimentation coefficients, ρ P =4.51 g cm −3 . With the particle density in hand, Equation 5b is utilized to calculate molecular weight, M =35,260±180 Da. Remarkably, the molecular weight predicted by theory for Au 144 (SR) 60 is M =36,597 Da, giving our method <4% error. The molecular weight found by ESI-MS [33] for the sample studied was M =36,598 Da. Finally, the ρ P and sedimentation coefficient are transformed into particle diameter ( d P ) by Equation 5c. The distribution of the diameters is weight-averaged to a single value after normalizing by the concentration distribution, d P =2.83±0.01 nm. 2D AUC of a mixture of monodisperse standard nanoclusters As a next step, we tested the validity of our method on a mixture of three atomically discrete thiolated gold NPs with the same type of organic ligand, also of exactly known molecular formula [33] , [34] , [35] , [36] , [37] , [38] . Again we obtain an excellent match (~2–3% error) between the actual molecular weights measured by ESI-MS and the ones we obtained with our method. Three Au nanocluster standards were mixed together: Au 25 (SR) 18 TOA, Au 38 (SR) 24 and Au 144 (SR) 60 ( R =−CH 2 CH 2 Ph). The Au 25 (SR) 18 TOA nanocluster was bound to a tetraoctylammonium ion (TOA + ) due to its negative monovalency [39] . After AUC, sedimentation coefficient distributions were fit to the experimental data with SEDFIT (σ=0.683), and the s - and D -distributions ( Fig. 3b ) were transformed into diameters, densities and molecular weights, by the same procedure used for the single Au 144 (SR) 60 nanoclusters. The 2D distributions can be integrated over all diffusion coefficients and reduced to a one-dimensional plot ( Fig. 3a ). Table 2 summarizes the 2D experimental data for the three NPs sedimented together in solution. 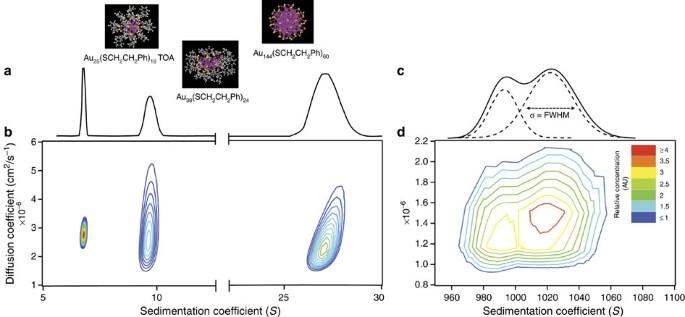Figure 3: 2D AUC distributions for both nanoclusters and PDT-capped nanoparticles. The three 'magic-sized' clusters were mixed in toluene (T=20 °C) and sedimented simultaneously, to illustrate the accuracy and ease of measuring sedimentation and diffusion coefficients for a distribution of species. (a) The integrated 1D sedimentation coefficient distribution over the respective values of diffusion coefficients. (b) 2D sedimentation and diffusion coefficient distributions for three thiolated gold nanoclusters. (c) The integrated one-dimensional distribution of sedimentation coefficients taken over all diffusion coefficients and the multi-peak Gaussian fit illustrating the resolution of two PDT-NP peaks. (d) The sedimentation and diffusion coefficient distributions for PDT-NPs. Figure 3: 2D AUC distributions for both nanoclusters and PDT-capped nanoparticles. The three 'magic-sized' clusters were mixed in toluene (T=20 °C) and sedimented simultaneously, to illustrate the accuracy and ease of measuring sedimentation and diffusion coefficients for a distribution of species. ( a ) The integrated 1D sedimentation coefficient distribution over the respective values of diffusion coefficients. ( b ) 2D sedimentation and diffusion coefficient distributions for three thiolated gold nanoclusters. ( c ) The integrated one-dimensional distribution of sedimentation coefficients taken over all diffusion coefficients and the multi-peak Gaussian fit illustrating the resolution of two PDT-NP peaks. ( d ) The sedimentation and diffusion coefficient distributions for PDT-NPs. Full size image Table 2 Data from the 2D AUC distributions for both nanoclusters and PDT-capped nanoparticles. Full size table Determination of particle composition In the very common case of a NP composed of two phases (for example, core–shell NPs and monolayer protected NPs) we can obtain a reasonable estimate of the composition of the particle by combining the measured M and ρ P with the bulk densities (usually tabulated or easily measured) of the two phases. For example, the values for the core and ligand densities [27] , [28] are: bulk gold: 19.32 g cm −3 ; bulk ligand: 1.03 g cm −3 . Combining mass conservation where N core and N shell represent the number of atoms in the core and the number of molecules in the shell, respectively, with an additive volume consideration: a set of equations is yielded that can be solved for N shell and N core , and thus molecular formula: For the Au 144 (SR) 60 nanoparticle, the estimated molecular formula by AUC was calculated with Equation 8 to be Au 137 (SR) 60 , a decent estimate of the actual molecular formula ( Table 1 ). Given instead the actual molecular formula, it is possible to back calculate (by Equation 8) the density of the ligand shell. For the Au 144 (SR) 60 nanocluster, the ligand shell density was found to be ρ L =1.2 g cm −3 , slightly higher than the bulk ligand density, as expected for these types of curved systems [28] . Table 1 Estimated molecular formula and ligand shell density for standard nanoclusters. Full size table 2D AUC of PDT-coated nanoparticles In order to prove the validity of our technique for large NPs, we applied the method to larger, pentadecanethiol gold nanoparticles (PDT-NPs) synthesized using the Stucky method (see Methods for details) [40] . These particles are illustrative of the often-encountered case of so-called 'nearly' monodisperse particles. The 2D sedimentation and diffusion plot for this sample is shown in Figure 3d . From this data we can extract the size, density and molecular weight of the sample, as outlined in previous paragraphs. Furthermore, we can use the bulk densities of the core ( ρ Au =19.32 g cm −3 ) and shell ( ρ PDT =0.85 g cm −3 ), to estimate the average molecular formula, the core diameter and the shell thickness. The data is summarized in Table 2 . Unlike the previous NP standards ( Fig. 3b ), the PDT-NPs, although narrowly dispersed, are not discrete species. This signifies that the standard deviation in core diameter is indicative of sample properties rather than the intrinsic instrumental broadening of the peaks. By transmission electron microscopy (TEM) ( Supplementary Fig. S2 ), the average core diameter ( d core ) and standard deviation of the PDT-NPs was 6.7±0.07 nm—essentially a perfect match with our AUC analysis. Yet our results reveal that AUC provides a more complete analysis as our results show that the core diameter is actually composed of a bi-modal distribution of nanoparticles, irresolvable with TEM, 6.68±0.10 nm and 6.82±0.06 nm. 2D AUC of polydisperse gold nanoparticles After proving the effectiveness of our technique for NPs of various sizes, we now demonstrate the power of our technique by characterizing truly polydisperse particles, the most general case encountered in unrefined nanoparticle systems. To this end, we tested a polydisperse sample of sodium 11-mercaptoundecanesulfonate-capped AuNPs (MUS-NPs). The core diameter distribution of these particles ranges from ~4–9 nm, as suggested by TEM ( Supplementary Fig. S2 ). The NPs were dissolved in 0.15 M NaCl and sedimented with AUC at 20 °C at a speed of 5,000 r.p.m. 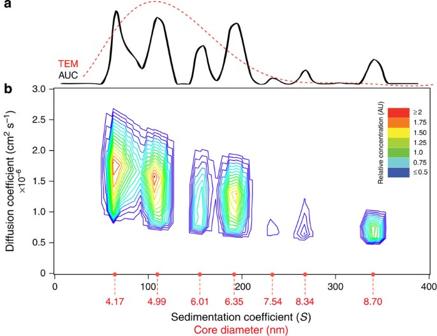Figure 4: 2D AUC distribution of polydisperse gold nanoparticles. (a) The integrated 1D distribution of sedimentation coefficients taken over all diffusion coefficients and the overlaid particle size distribution by TEM, to illustrate the increase in resolution by AUC. (b) The sedimentation and diffusion coefficient distributions for the polydisperse NP sample. The 2D sedimentation and diffusion plot for this sample is shown in Figure 4 . Figure 4: 2D AUC distribution of polydisperse gold nanoparticles. ( a ) The integrated 1D distribution of sedimentation coefficients taken over all diffusion coefficients and the overlaid particle size distribution by TEM, to illustrate the increase in resolution by AUC. ( b ) The sedimentation and diffusion coefficient distributions for the polydisperse NP sample. Full size image The molecular weights, densities and hydrodynamic diameters obtained by 2D SV-AUC are in extremely good agreement with the theoretical and experimental data in the literature for those clusters, and were all obtained in solution with a single experiment. Parameters are reported to three significant digits, because the radial positions and solvent density are known accurately to the same significance. A comparison between the cluster's sedimentation behavior when run alone compared to when it was run together with the other clusters revealed no statistically significant difference ( t -test, σ=0.95) in the measured s and D values of the nanoclusters between both situations. We notice that the errors for the parameters determined for the three clusters vary between the three types. Even though they slightly increase with the cluster size at this point, we believe that the error is related to the non-ideality in the shape of the nanocrystals. Indeed, according to crystallographic data, Au 25 (SR) 18 TOA is quasi-spherical with an aspect ratio very close to 1, whereas A 38 (SR) 24 is rod-like with an aspect ratio of ~1.3 (refs 35 , 39 ). It is, therefore, not surprising that the error in molecular weight for Au 38 (SR) 24 is slightly higher compared with Au 25 (SR) 18 TOA, because the basis of our analysis is the validity of Stoke's Law for describing the diffusion of the particles. The encouraging results obtained from the nanoparticle standards open the possibility of applying the 2D SV-AUC method outlined above to naturally polydisperse samples, which exhibit dispersity in size, density and molecular weight. In this way, we are able to examine a particular population in a distribution, without requiring homogeneity in density (typically required in AUC experiments). These results also confirm that our methodology is robust enough to handle NPs that deviate from the spherical-shape requirement in Stokes Law (Equation 3); as the NPs in Figure 3b are known to be highly faceted or slightly prolate [35] , [39] . Yet, one should not push this concept too far. In samples with particles with widely varying aspect ratios, it would not be possible to apply our method without a priori knowledge on the aspect ratio of the specific (fractionated) populations. For example, the application of our method to analyse nanorods requires the knowledge of their aspect ratio. Equation 8 was used to approximate the molecular formulas and ligand shell densities ( Table 1 ), given the bulk core/ligand densities and theoretical molecular formulas. The estimated molecular formulas for the three NP standards confirm that the bulk ligand density could be used to reasonably approximate the actual ligand shell density. On the other hand, if prior knowledge of the molecular formula is available, one may be interested in using our methodology to measure the density of the ligand shell, as illustrated in Table 1 . It should be noted that nanoparticles in the size range of the PDT-NP sample ( Fig. 3d ), or larger, have small diffusion coefficients and typically sediment quickly, hence care must be taken in the choice of rotor speed. The general approach is to decrease the speed to increase the influence of diffusion during sedimentation while still maintaining sedimentation as the dominant transport mechanism. This yields a more accurate measurement of the diffusion coefficient, without compromising precision in the measurement of the sedimentation coefficient. In other words, a slower speed is necessary to accurately observe the diffusion of larger nanoparticles. The time scale of the experiment, however, remains only a few hours and still just a single run is required. Further work will be needed to determine a precise criterion to determine the optimal speed for a given sample. For the sample of polydisperse MUS-coated NPs, the core diameter was calculated from the 2D sedimentation and diffusion plot and presented in Figure 4b . The core diameter distribution obtained by TEM was qualitatively overlaid onto the 1D AUC plot in Figure 4a to illustrate the level of resolution unobtainable by TEM, even when combined with other techniques. Even though the core size distributions show a good overall agreement in size range, 2D SV-AUC reveals the presence of distinct populations in the sample that are obscured by the comparatively tiny sampling capability of TEM. Previously, Colfen et. al. have demonstrated the angstrom resolution of AUC analysis and its potential power in replacing other lower-resolution techniques [41] . SV-AUC distributions sample millions to billions of particles [23] , wheras TEM histograms can accommodate a few thousand particles at most. Given this level of detail, it should be immediately obvious to the reader that SV-AUC could be a powerful tool to understand nanoparticle growth [24] . Also, the core diameter distributions are the only parameters easily obtained by TEM. Even though insight into the ligand shell is in theory possible with advanced high-angle annular dark-field scanning transmission electron microscopy [42] , the technique is not practical for statistically assessing its properties, especially in an industrial setting. In a single experiment, our method provides the core size, overall particle diameter, and density for each population of NPs present in our sample without the need for a global analysis. As well as the shape variations described in previous sections, charges on nanoparticles can also lead to non-ideality. The MUS-coated particles described above were prepared in salt solutions to screen the highly charged surface (zeta potential (ζ)=−38±5.30 mV) [8] . The classical way to measure whether electrostatic gradients induced by centrifugation affect the sedimentation coefficient of a sample is to run the solute in a series of solutions differing in ionic strength [23] . Provided that one can accurately measure the density and viscosity of the ionic buffer solution, the application of our method can be applied to highly charged solutes. We believe that our method has general applicability, even beyond nanoparticles; yet, we do acknowledge limitations for our approach. First, some non-ideal samples would require assumptions. For example, the analysis of rods with varying shape should be coupled with another sizing technique to predetermine the aspect ratio. For a solute which is relatively monodisperse in axial ratio, our analysis could be applied with little adaptation. Recent developments in multi-wavelength AUC by Colfen et al . could prove excellent for this type of sample by providing a third axis of information that could be used to eliminate the need for prior axial ratio determination [43] . Alternatively, preparative fractionation prior to AUC could significantly reduce the complexity of the solute. Future work by our group will explore this possibility. Other types of non-ideality could be samples with widely varying charge density, or with density varying with size, but in unpredictable ways. Moreover, the sample shown in Figure 4 is actually composed of nicely discrete population of particles; this helps to reduce the error in our analysis. Samples with continuously varying sedimentation coefficient distribution, such as polymers or polymer-coated nanoparticles, would require an artificial binning of the data that would introduce another source of error. For example, we tried to determine the iron content of ferritin type-I and found that we needed a set of additional assumptions to achieve a qualitative description of the complex [44] , [45] . The 2D SV-AUC NP characterization approach described herein provides unprecedented access to the size, density and molecular weight distributions of NPs, from a single experiment and without the use of standards or auxiliary measurements—as is usually required for quantitative characterization with AUC. We proved the accuracy and the generality of our approach by testing NPs of various size distribution modes (for example, mixtures of atomically discrete particles, narrowly dispersed particles and polydisperse particles of a wide size distribution). We find that our approach delivers precise insight into the density, molecular weight and size distributions. Furthermore, no burdensome or speculative global analysis is needed to correlate these property distributions to one another—as is required when one studies different sample properties with multiple characterization methods. Even though our methodology relies on Stokes' law to derive the various property distributions of NPs, we find that it is robust enough to handle NPs that slightly deviate (for example, oblate and faceted) from the spherical shape assumption of Stokes' law (formulated for a hard-sphere in a continuum liquid). Furthermore, we were able to accurately measure the properties of some of the smallest NPs that can be presently synthesized ( d p ~2 nm) and thus exist in the regime of dominant intermolecular forces where Stokes' law is expected to break down. This discovery is of great importance to anyone interested in techniques that rely on Stokes' law for particle sizing (for example, dynamic light scattering (DLS), FFF and electrophoresis) and nanorheolgy in general. NP research has seen an upsurge in size fractionation techniques in recognition of the need to minimize heterogeneity in NP samples that are intended for various applications. The methodology demonstrated in this work is ideally suited to work hand-in-hand with this trend, because it simultaneously maps a particle's density, size and molecular weight to its s and D values. Therefore, it provides not only the properties of the NPs present in a given sample, but also a solution allowing researchers to select (that is, fractionate) species in the sample based on pre-desired properties: a technique we are currently developing for future work. We believe this advantage, in addition to the accuracy, ease and general nature of our 2D SV-AUC treatment, will render this technique indispensible for the future studies and applications for all types of core–shell NPs. Analytical ultracentrifugation AUC was performed using a Beckman Optima XL-A, An-60 Ti rotor, scanning absorbance optics, with 12-mm path length double sector centerpieces with sapphire windows. Epon centerpieces were used for water (MUS-NPs) and hexanes (PDT-NPs), and aluminum centerpieces for samples in toluene (NCs). All measurements were made at 520 nm, 20 °C, at speeds ranging from 3,000 r.p.m. to 40,000 r.p.m. and data ranges from over 50–100 scans were chosen to be representative of the whole run (radial step size of 0.003–0.008 cm). SV runs typically required 0.05 to 0.5 mg of material in 400 μL solution. Each sample was prepared at varying concentrations to ensure that the sedimentation and diffusion coefficients were not concentration dependent. An inhomogeneous solvent model was applied to account for solvent compressibility caused by high pressure build-ups at the centrifugal fields obtained at high rotor speed [23] . The sedimentation and diffusion coefficients are provided under normal conditions (20 °C, water) and must be converted to the appropriate solvent [46] . Measurement of AUC experimental error To obtain a measure of the experimental standard deviation of AUC, the Au 144 (SR) 60 NP was repeatedly measured a total of 10 times at 20 °C in toluene at 8,000 r.p.m. The results were extraordinarily reproducible in both s and D , measured to be: 27.1±0.1 S and (2.5±0.1)×10 −6 cm 2 s −1 , respectively. Hence, for both cases the standard deviation is limited by the line width we measure for a single experiment (~4% of the average). To compare the difference between AUC analysis of the standard nanoclusters sedimented separately and together, a t -test was used (σ=0.95), assuming the data was normally distributed (visual test). For a grid of 10 f / f 0 values and 30 s values, the degrees of freedom n =300. Synthesis of Au 25 (SC 2 H 4 Ph) 18 TOA nanoclusters HAuCl 4 ·3H 2 O (0.4 mmol) was dissolved in 5 ml Nanopure water, and tetraoctylammonium bromide (TOAB, 0.47 mmol) was dissolved in 10 ml toluene; the two solutions were combined and vigorously stirred to facilitate phase transfer of Au(III) salt into the toluene phase. After phase transfer was completed, the aqueous phase was removed using a glass pipette. The toluene solution of Au(III) was cooled to 0 °C in an ice bath over a period of 30 min under constant magnetic stirring. PhC 2 H 4 SH (~3 equivalents per mole of gold) was added and stirring was reduced to a very low speed. The deep red solution turned faint yellow over a period of ~5 min, and finally clear over ~1 h. After that, the stirring speed was changed to fast stirring (~1100 r.p.m.) and, immediately, an aqueous solution of NaBH 4 (4 mmol, 10 equivalents per mole of gold, freshly made in 7 ml ice-cold nanopure water) was rapidly added all at once. The reaction was allowed to proceed overnight. Then the aqueous layer at the bottom of the flask was removed and the toluene solution was dried on a rotary evaporator. Ethanol or methanol was added to separate Au 25 clusters from TOAB and side products (for example, disulfide), and so on. Pure Au 25 clusters were collected by extracting with acetonitrile [38] . Synthesis of Au 38 (SC 2 H 4 Ph) 24 nanoclusters In a typical experiment, 0.5 mmol HAuCl 4 ·3H 2 O and 2.0 mmol glutathione powders were mixed in 20 ml acetone at room temperature under vigorous stirring for ~20 min. The mixture (yellowish cloudy suspension) was then cooled to ~0 °C in an ice bath. After ~20 min, a solution of NaBH 4 (5 mmol, dissolved in 6 ml ice-cold nanopure water) was rapidly added to the suspension under vigorous stirring. The solution colour immediately turned black after addition of NaBH 4 , indicating the formation of Au nanoclusters. After ~20 min, black Au n (S G ) m nanoclusters precipitated out of the solution and deposited onto the inner wall of the flask, leaving a clear acetone solution. The clear solution was then decanted and 6 ml water was added to dissolve the Au n (S G ) m clusters. A solution of Au n (S G ) m (around 200–300 mg, dissolved in 6 ml nanopure water) was mixed with 0.3 ml ethanol, 2 ml toluene and 2 ml PhC 2 H 4 SH. Note that ethanol is added to prompt phase transfer of Au n (S G ) m from water to organic phase. The diphase solution was heated to 80 °C and maintained at this temperature, under air. The Au n (S G ) m clusters were found to transfer from the water phase to the organic phase in less than 10 min. The thermal process was allowed to continue for ~40 h at 80 °C. Over the long etching process, the initial polydisperse Au n nanoclusters were finally converted to monodisperse Au 38 (SC 2 H 4 Ph) 24 clusters. The Au clusters were precipitated and washed thoroughly with ethanol (or methanol) to remove excess thiol. Then, the Au 38 (SC 2 H 4 Ph) 24 nanoclusters were simply separated from Au(I)-S G (poorly soluble in almost all solvents) by extraction with dichloromethane or toluene [36] . Synthesis of Au 144 (SC 2 H 4 Ph) 60 nanoclusters HAuCl 4 ·3H 2 O (0.45 mmol) was dissolved in 5 ml nanopure water, and TOAB (0.52 mmol) was dissolved in 10 ml toluene. After mixing, the solution was vigorously stirred until phase transfer of Au(III) was completed (the toluene phase became deep red, whereas the initial yellow aqueous phase became clear). The clear aqueous phase was removed using a 10 ml syringe. The toluene phase containing Au(III) were cooled to 0 °C in an ice bath for ~30 min. Then, PhC 2 H 4 SH (~ 3 equivalents of Au) was added under fast magnetic stirring. The deep red solution turned yellow gradually and finally almost clear in ~1 h. NaBH 4 solution (4.5 mmol, dissolved in 5 ml ice-cold nanopure water) was rapidly added to solution all at once. The solution colour immediately changed to black. The reaction was allowed to proceed for ~24 h. After ~24 h, the aqueous phase was discarded and the black toluene phase was dried by rotary evaporation. Ethanol was used to separate the Au nanoclusters from TOAB and other side products. To obtain truly monodisperse Au 144 nanoclusters, excess PhCH 2 CH 2 SH was used to etch the as-prepared Au nanoclusters from the first step. Typically, 20 mg Au nanoclusters was dissolved in 1 ml toluene, and 0.5–0.8 ml neat PhC 2 H 4 SH was then added to the Au nanoclusters solution. The solution was heated to 80 °C and maintained at 80 °C for about 24 h under constant magnetic stirring. After that, 20 ml methanol was added to the solution to precipitate Au nanoclusters. Only Au 144 nanoclusters and Au(I)-SCH 2 CH 2 Ph exist in the black precipitation. Au 144 nanoclusters were extracted with CH 2 Cl 2 , and Au(I)-SCH 2 CH 2 Ph residuals (poorly soluble) were discarded [33] . Molecular weight determination of nanoclusters Electrospray ionization (ESI) mass spectra were used to determine the molecular weight of Au 25 (SC 2 H 4 Ph) 18 − TOA + , Au 38 (SC 2 H 4 Ph) 24 and Au 144 (SC 2 H 4 Ph) 60 nanoclusters (the latter two clusters are charge neutral) (see Supplementary Fig. S3 ). ESI mass spectra were recorded using a Waters Q-TOF mass spectrometer equipped with Z-spray source. The source temperature was kept at 70 °C. The sample was directly infused into the chamber at 5 μl min −1 . The spray voltage was kept at 2.20 kV and the cone voltage at 60 V. The ESI sample was dissolved in toluene (1 mg ml −1 ) and diluted (1:2 vol) by dry methanol (containing 50 mM CsOAc to enhance cluster ionization in ESI). The experimental error of formula weight determination is typically <0.3 Da (within the range of <10,000 Da). Synthesis of pentadecanethiol gold nanoparticles 0.25 mmol chlorotriphyenylphosphine gold (AuPPh 3 Cl) was mixed with 0.75 mmol PDT in 20 ml of benzene to form a clear solution, to which 2.5 mmol of tert-butyl amine borane complex was then added. The mixture was stirred at 55 °C for 1 h, and then cooled to room temperature. 100 ml of ethanol was then added to precipitate the NPs. The precipitated NPs were collected by centrifugation and washed three times with a mixture of benzene and ethanol. The highly reproducible monodisperse NPs were obtained without any further treatment [40] . How to cite this article: Carney, R.P. et al . Determination of nanoparticle size distribution together with density or molecular weight by 2D analytical ultracentrifugation. Nat. Commun. 2:335 doi: 10.1038/ncomms1338 (2011).